Sponges with covalently tethered amines for high-efficiency carbon capture Adsorption using solid amine sorbents is an attractive emerging technology for energy-efficient carbon capture. Current syntheses for solid amine sorbents mainly based on physical impregnation or grafting-to methods (for example, aminosilane-grafting) lead to limited sorbent performance in terms of stability and working capacity, respectively. Here we report a family of solid amine sorbents using a grafting-from synthesis approach and synthesized by cationic polymerization of oxazolines on mesoporous silica. The sorbent with high amount of covalently tethered amines shows fast adsorption rate, high amine efficiency and sorbent capacity well exceeding the highest value reported to date for low-temperature carbon dioxide sorbents under simulated flue gas conditions. The demonstrated efficiency of the new amine-immobilization chemistry may open up new avenues in the development of advanced carbon dioxide sorbents, as well as other nitrogen-functionalized systems. Rising levels of atmospheric CO 2 due to increasing consumption of fossil fuels have been widely implicated as a critical factor contributing to global climate change [1] . Post-combustion carbon capture and storage (CCS) approaches based on retrofitting the existing energy infrastructure provide a viable near-term solution to reduce anthropogenic CO 2 emissions. The current benchmark carbon-capture technology, amine scrubbing, is based on CO 2 absorption using liquid amine solutions. Despite great advances in process optimization, this technology suffers from issues associated with the use of amine solutions such as equipment corrosion, solvent loss and toxicity and requires extensive energy for sorbent regeneration [2] . In this regard, CO 2 adsorption using solid amine sorbents has been proposed as an attractive alternative for post-combustion carbon capture [3] , [4] , [5] , [6] , [7] , [8] , [9] , [10] , [11] , [12] , [13] , [14] , [15] , [16] . As amine molecules are immobilized onto the solid sorbent supports, the issues associated with the use of liquid amines can be minimized. Moreover, the much lower heat capacities of solid sorbents may significantly reduce the energy penalty related to sorbent regeneration. Furthermore, amine sorbents show high selectivity towards CO 2 even in the presence of moisture, making them applicable to CCS for low-pressure, dilute CO 2 exhausts, in contrast to common physical adsorbents such as zeolites, activated carbons and more recently many metal-organic frameworks (MOFs) that show great promise but typically work in dry CO 2 at moderate or high partial pressures. Presently, most of the advanced amine sorbents utilize porous materials, particularly mesoporous silicas, as supports on which amines are immobilized physically via wet impregnation [4] , [6] , or covalently either by post-grafting [10] , [17] or cocondensation of aminosilanes and tetraalkoxysilanes [16] . These amine sorbents exhibit attractive CO 2 -capture properties including fast adsorption kinetics and low operating temperatures. However, challenges remain before they can be adopted for practical CCS applications. A major problem lies in insufficient working capacity. Current amine sorbents typically contain relatively low amine functionality and show limited amine efficiency (the stoichiometric ratio of captured CO 2 to amine immobilized on the sorbents). An increase in the amine content usually comes at the expense of amine efficiency, because of blocking of active sites ultimately compromising sorbent performance. Consequently, most of solid amine sorbents exhibit CO 2 capacities <4 mmol g −1 under flue gas conditions, barely approaching the capacity threshold to economically compete with the liquid amine-scrubbing process [18] . In addition to sorbent capacity, long-term stability under flue gas conditions, especially for sorbents based on impregnated amines, is also a concern. A promising solution involves immobilizing amines on sorbent supports via strong chemical bonds to improve sorbent stability and cycling performance. Therefore, intensive efforts have been devoted to developing high-efficiency sorbents with covalently attached amines. However, most of the previous studies have mainly focused on the optimization of the sorbent support structure, with few reports advancing the chemistry to enhance the amine/support ratio as well as the amine efficiency of the sorbents [5] , [19] , [20] . Stepwise growth of melamine dendrimers and ring-opening polymerization of Z-protected L -lysine N -carboxyanhydride have been used previously to improve the amount of amine content [20] , [21] , [22] . Unfortunately, the available amine groups for CO 2 in these sorbents are relatively low leading to limited sorbent performance. A notable advance was recently achieved by Jones et al . [5] , where a new family of aminosilica sorbents with covalent tethering of hyperbranched polyamines has been synthesized via in situ polymerization of aziridine [23] . These sorbents exhibit high CO 2 capacities up to 5.6 mmol g −1 and good sorbent stability after 11 adsorption–desorption cycles under controlled gas conditions (humidified 10% CO 2 with ~1.6% water) [5] , [23] . However, despite the notable performance improvements, the yield of the grafted polyamines is relatively low (<40%) when the ratio of aziridine to the support is high, and the amine loading is limited to <9.8 mmol N g −1 (ref. 23 ). The amine efficiency drops with increasing amine loadings (CO 2 /N<0.6, when the amine loading is above 7 mmol N g −1 ), probably due to the uncontrolled polymerization of aziridine outside the silica support [24] . Here we report an approach for the synthesis of high-efficiency CO 2 sorbents with covalently tethered polyamines via grafting-from cationic polymerization of oxazolines. The new class of CO 2 sorbents exhibits the highest ever amine content (over 15 mmol N g −1 ) well exceeding any covalently functionalized supported amine sorbents reported previously. The sorbents exhibit an exceptional amine efficiency (CO 2 /N>0.8) even at high amine loadings, leading to an outstanding capacity (~12 mmol g −1 ) under simulated flue gas conditions (8% CO 2 with a relative humidity of 18% at 25 °C). To the best of our knowledge, this is the first report for a low-temperature sorbent showing CO 2 capacity above 8 mmol g −1 , with demonstrated stability in humid dilute CO 2 (see Supplementary Fig. 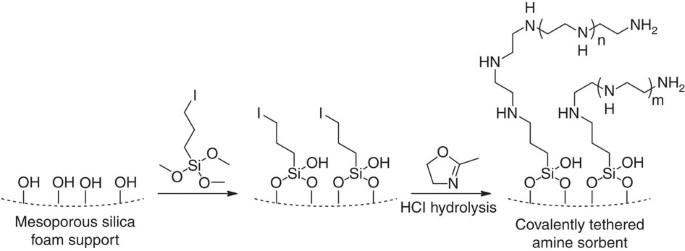Figure 1: Schematic showing the synthesis of the covalently tethered amine sorbent. The synthesis involves grafting alkyliodine as the initiator, followed by growing the amino polymer on the mesoporous support via the cationic polymerization of 2-methyl-2-oxazoline and finally acid hydrolysis to produce the polyethylenimine-tethered sorbent. 1 and Supplementary Table 1 for sorbent performance comparisons of main classes of sorbents with typical working temperature below 150 °C). As the amine-immobilization chemistry is simple with no highly toxic or expensive chemicals involved, and more importantly, the versatility to tailor the molecular architecture of the grafted amine-containing polymers [25] , we believe this method can be further extended to a wide range of systems including advanced functional membranes, drug-delivery vehicles and basic catalysts. Synthesis of the CO 2 sorbent Figure 1 illustrates the synthesis approach, which involves functionalizing a mesoporous silica foam [26] with alkyliodine to initiate the growth of linear polyethylenimine (PEI) on the sorbent support. The surface iodination of the silica support was corroborated via X-ray photoelectron spectroscopy (XPS). Two distinctive XPS peaks at 621 and 633 eV for I 3d5/2 and I 3d3/2 , respectively, ( Supplementary Fig. 2 ) were observed for the silica support after functionalization with 3-iodopropyltrimethoxysilane, which can be attributed to the I–C bond of the silane. The presence of linear PEI was confirmed via Fourier transform infrared (FTIR) and nuclear magnetic resonance (NMR) analyses ( Supplementary Figs 3–5 ). Briefly, the vibrations at 3,217 and 1,616 cm −1 in the FTIR spectrum correspond to the symmetric stretching and bending vibration of N–H, respectively. The strong resonance at 50.4 p.p.m. in the cross-polarization magic-angle spinning 13 C NMR spectrum can be assigned to the carbons in the repeat unit (– C H 2 – C H 2 –NH–) of PEI. Finally, the inversely gated 13 C NMR spectrum of the polymer cleaved from the sorbent shows two resonance peaks at 49.1 and 41.3 p.p.m. attributed to the carbons from the –NH– C H 2 – C H 2 –NH– and NH 2 – C H 2 –CH 2 –NH– units of PEI, respectively, indicating that the polymer molecules grafted on the silica support are essentially linear PEI. The number average molecular weight of the linear PEI estimated from the relative intensity of the two NMR peaks is about 1,010, consistent with the results from Matrix-assisted laser desorption/ionization time-of-flight mass spectrometry (MALDI-TOF MS) ( Supplementary Fig. 6 ). Figure 1: Schematic showing the synthesis of the covalently tethered amine sorbent. The synthesis involves grafting alkyliodine as the initiator, followed by growing the amino polymer on the mesoporous support via the cationic polymerization of 2-methyl-2-oxazoline and finally acid hydrolysis to produce the polyethylenimine-tethered sorbent. Full size image The key advance for the sorbent design here is the growth of polyoxazoline via cationic polymerization of oxazolines [25] , where the amine polymers propagate progressively from the support surface. Therefore, a relatively uniform amine coating inside the mesopores, allowing a high content of covalently tethered amines with minimized blocking to the hierarchical structure of the support, could be achieved leading to superior sorbent performance. The structure and morphology of the sorbent was investigated via transmission electron microscopy (TEM), scanning electron microscopy (SEM) and nitrogen adsorption measurements. The pristine sorbent support ( Fig. 2a,c ) shows a hierarchical structure of interconnected large macropores (from hundreds of nanometres to microns) while the silica framework is composed of cells with sizes in the range of 40–80 nm. As seen from the SEM image in Fig. 2b , the cells of the sponge-like amine sorbent appear to have a relatively uniform coating layer of amine polymers, as supported by the elemental mapping ( Supplementary Fig. 7 ). The TEM image in Fig. 2d further confirms the grafting of amine polymers in the mesoporous unit cells. It should be noted that after the amine functionalization, the hierarchical porous structure largely remains, which facilitates CO 2 diffusion inside the sorbent improving the amine efficiency and adsorption rate. 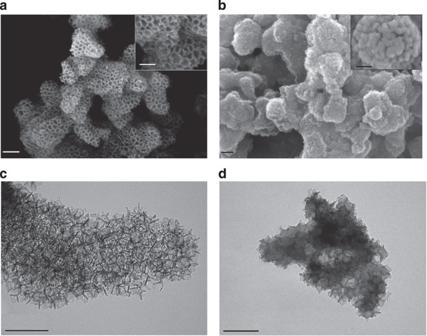Figure 2: Structure of the pristine silica support and the amine sorbent. (a) SEM image of the pristine silica support. (b) SEM image of the amine sorbent. (c) TEM image of the pristine silica support. (d) TEM image of the amine sorbent. Scale bars, 200 nm for the main images, and 100 nm for the images in the inset. Figure 2: Structure of the pristine silica support and the amine sorbent. ( a ) SEM image of the pristine silica support. ( b ) SEM image of the amine sorbent. ( c ) TEM image of the pristine silica support. ( d ) TEM image of the amine sorbent. Scale bars, 200 nm for the main images, and 100 nm for the images in the inset. Full size image The nitrogen adsorption of both the pristine silica support and the amine sorbent follow a type IV isotherm with a hysteresis loop starting at high relative pressures of around 0.85 ( Fig. 3 ). The calculated Brunauer–Emmett–Teller (BET) surface area and the total pore volume of the pristine support, using the simplified Broekhoff-de Boer method [27] , are 498 m 2 g −1 and 2.69 cm 3 g −1 , respectively. In contrast, the corresponding values for the amine sorbent decrease to 23.4 m 2 g −1 and 0.044 cm 3 g −1 , respectively. These nitrogen adsorption data imply that most of the sponge-like cells of the support are largely occupied by the amine molecules, consistent with the results from the SEM and TEM images in Fig. 2 . 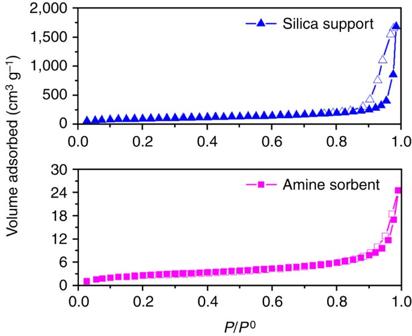Figure 3: Nitrogen sorption isotherms. Nitrogen sorption isotherms of the pristine silica foam support and the amine sorbent at 77 K. The solid and open symbols represent adsorption and desorption, respectively. Figure 3: Nitrogen sorption isotherms. Nitrogen sorption isotherms of the pristine silica foam support and the amine sorbent at 77 K. The solid and open symbols represent adsorption and desorption, respectively. Full size image CO 2 adsorption of the sorbent The adsorption of the amine sorbent in dilute CO 2 (8% dry CO 2 or a simulated flue gas containing 8% CO 2 with a relative humidity of 18% at 25 °C) was investigated using the Q500 thermal gravimetric analyzer system, as illustrated in Supplementary Fig. 8 . It is worth noting that the amine sorbent may adsorb moisture from humid gases because of its highly hydrophilic nature. Therefore, prior to CO 2 adsorption in the simulated flue gas, the sorbent was equilibrated to a constant weight in N 2 with the same moisture level as the CO 2 gas to minimize potential errors associated with moisture adsorption in the adsorption measurements ( Supplementary Fig. 9 ) [28] . As shown in Fig. 4a , a fast CO 2 uptake occurred once the sorbent was exposed to CO 2 , followed by a gradually slower adsorption process. Such two-stage adsorption behaviour is typical of many amine adsorbents [3] , [4] , [12] and has been attributed to increasing CO 2 diffusion resistance during adsorption [3] , [4] , [5] , [13] . Interestingly, the sorbent showed distinct adsorption behaviour in dry CO 2 comparing with that in the simulated flue gas, despite the same CO 2 concentration level. In dry 8% CO 2 , the sorbent showed limited adsorption ~0.82 mmol g −1 at 25 °C after 120 min, whereas a much higher CO 2 capacity up to 4.30 mmol g −1 with noticeable faster CO 2 uptake rate at the first stage of adsorption was observed at 60 °C. We attribute the higher capacity to the lower CO 2 diffusion resistance due to higher flexibility of the immobilized polyamine molecules at the elevated temperature. In sharp contrast, in the simulated flue gas the sorbent exhibited fast CO 2 adsorption at 25 °C and the capacity of the sorbent reached ~11 mmol g −1 in the first 30 min (and up to 11.8 mmol g −1 by 120 min), which is about twice the previous capacity records of other amine sorbents [23] and MOFs [29] under simulated flue gas conditions ( Supplementary Fig. 1 ), and about 9 times higher the capacity of amine-scrubbing solutions (for example, ~1.25 mmol g −1 for 30% monoethanolamine solution [30] ). Further comparing the adsorption behaviour of the sorbent in dry CO 2 and in simulated flue gas at 60 °C, it is clear that the presence of moisture significantly improves the CO 2 -capture performance of the sorbent. Since the N content of the sorbent determined via elemental analysis is ~15.1 mmol N g −1 , the amine efficiency (CO 2 /N) of the sorbent at 25 °C for 120 min is ~0.8, among the highest reported for amine sorbents even at such high amine content [3] . It should be noted that since the sorbent capacity kept increasing after 120 min, the final amine efficiency (CO 2 /N) of the sorbent could be even higher. This result is in sharp contrast to other supported amine sorbents with high amine loadings such as the sorbents prepared via wet impregnation and polymerization of aziridine, which show much lower amine efficiency (CO 2 /N=0.2~0.6) under their optimal adsorption conditions [23] , [24] , [26] . The high amine efficiency observed here could be partially attributed to the optimized hierarchical structure of the sorbent as well as the reaction mechanism of amine and CO 2 , where the formation of bicarbonates in the presence of moisture rather than carbamates in dry CO 2 theoretically enhances the efficiency of the primary and secondary amines from 0.5 to 1. In addition, the adsorbed water may serve as a plasticizer lowering the CO 2 diffusion resistance and further improving the amine efficiency [31] . 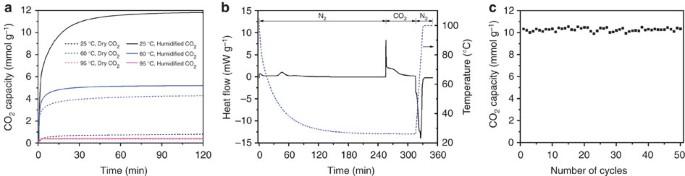Figure 4: Sorbent performance. (a) CO2adsorption kinetics of the sorbent at different temperatures in 8% CO2. (b) DSC profile of the sorbent during equilibration in humid N2, adsorption in humid 8% CO2for 60 min at 25 °C and desorption in humid N2at elevated temperatures. Both the N2and CO2gases were humidified at 25 °C by passing through a water saturator. (c) cyclic performance of the amine sorbent under simulated flue gas conditions. In a typical cycle, the activated sorbent was exposed to humid 8% CO2(20 ml min−1) at 25 °C for 30 min. After the adsorption step, the sorbent was heated to 100 °C and completely regenerated within 15 min in humid N2(20 ml min−1). The sorbent was then cooled down to 25 °C and equilibrated in humid N2to a constant weight prior to the next adsorption cycle. Figure 4: Sorbent performance. ( a ) CO 2 adsorption kinetics of the sorbent at different temperatures in 8% CO 2 . ( b ) DSC profile of the sorbent during equilibration in humid N 2 , adsorption in humid 8% CO 2 for 60 min at 25 °C and desorption in humid N 2 at elevated temperatures. Both the N 2 and CO 2 gases were humidified at 25 °C by passing through a water saturator. ( c ) cyclic performance of the amine sorbent under simulated flue gas conditions. In a typical cycle, the activated sorbent was exposed to humid 8% CO 2 (20 ml min −1 ) at 25 °C for 30 min. After the adsorption step, the sorbent was heated to 100 °C and completely regenerated within 15 min in humid N 2 (20 ml min −1 ). The sorbent was then cooled down to 25 °C and equilibrated in humid N 2 to a constant weight prior to the next adsorption cycle. Full size image To better understand the adsorption behaviour of the sorbent, CO 2 adsorption was further studied in the simulated flue gas using the packed-bed system illustrated in Supplementary Fig. 8 . The sorbent exhibited a fast CO 2 uptake of about 7.3 and 9.0 mmol g −1 after 30 and 60 min, respectively, at 25 °C ( Supplementary Fig. 10 ). The sorbent capacity approached a plateau of ~12 mmol g −1 after 300 min at 25 °C, consistent with the sorbent capacity measurements using the thermal gravimetric analysis (TGA) system. The sorbent also exhibited a fast desorption and was fully regenerated at 100 °C within 30 min in the packed bed. Recall that the sorbent capacity measured via TGA decreases significantly from ~12 to ~0.43 mmol g −1 as the temperature increases within a narrow temperature range from 25 to 95 °C ( Fig. 4a ), suggesting that the sorbent can be easily regenerated in the simulated flue gas at relatively low temperatures (below 100 °C), which is very beneficial for reducing the energy penalty for sorbent regeneration. Energy consumption for sorbent regeneration The reaction heat of the sorbent in 8% CO 2 with a relative humidity of 18% at 25 °C and the energy consumption for sorbent regeneration were monitored via a differential scanning calorimeter (DSC) [18] , [26] . As shown in Fig. 4b , once the sorbent was exposed to CO 2 a sharp positive heat-flow spike followed by a large broad DSC peak was observed, which can be attributed to the exothermic reaction of the tethered PEI with CO 2 seen in the adsorption studies. Integration of these peaks gives an adsorption heat of ▵ H r ~74.6 kJ mol −1 CO 2 , which is in the same range as those observed for other amine sorbents (~45–95 kJ mol −1 CO 2 ) [10] , [18] , [32] , [33] , but higher than those of other sorbents such as zeolites, activated carbons and MOFs (~30 to 50 kJ mol −1 CO 2 ) [32] , [34] , [35] , where physisorption is the principal mechanism, indicating that chemisorption plays a predominant role in our sorbent. To regenerate the sorbent, the gas was switched from CO 2 to N 2 with the same humidity level and the temperature was raised from 25 to 100 °C. Multimodal endothermic peaks were observed and the total energy required for sorbent regeneration was ~135 kJ mol −1 CO 2 , which is higher than those of certain supported amine sorbents exposed to dry CO 2 gas [26] . This is probably the result of the additional energy consumption to desorb the adsorbed moisture. Nevertheless, the regeneration energy penalty for the sorbent is still much lower than that for stripping 30% monoethanolamine solution (~209 kJ mol −1 CO 2 ) [36] . In fact, as the capacity of the sorbent is about 9 times higher than 30% monoethanolamine solution (~1.25 mmol g −1 ), much fewer adsorption–desorption cycles are required for the sorbent to capture the same amount of CO 2 , which may greatly reduce the overall energy consumption by cutting down the auxiliary energy penalty associated with pumping and transportation. Sorbent stability Robust long-term sorbent stability and short process cycle time are critical to lower cost in practical CO 2 -capture applications. Here a repetitive adsorption–desorption test under simulated flue gas conditions was used to evaluate the stability of the sorbent. In each adsorption–desorption cycle, the sorbent was first equilibrated to a constant weight in humid N 2 (relative humidity ~18%) at 25 °C and then exposed to humid 8% CO 2 (relative humidity ~18%) at 25 °C for 30 min, followed by desorption in humid N 2 (relative humidity ~18% at 25 °C) at 100 °C for 15 min. As shown in Fig. 4c , no loss of sorbent capacity was observed after 50 cycles under the testing conditions. To further examine the sorbent stability, the sorbent was aged under accelerated conditions in steam/air at 106 °C for 48 h. After being treated under these harsh conditions, the sorbent maintained a capacity of 7.2 mmol g −1 in the simulated flue gas ( Supplementary Fig. 11 ), still well above the reported capacity records of other types of supported amine sorbents [3] . The performance loss of the sorbent under these harsh accelerated aging conditions may be attributed to the oxidative degradation of the amines, and structural changes of the support [37] , [38] , [39] , as suggested by the slightly lower BET surface area of the sorbent after the treatment ( Supplementary Fig. 11 ). In summary, we have demonstrated a new approach, based on grafting-from cationic polymerization of oxazolines, for the synthesis of CO 2 sorbents containing high content of covalently tethered polyamines. The sorbent maintained high amine efficiency for CO 2 capture (>0.8) with a very high amine content (>15 mmol N g −1 ), leading to a record-high CO 2 capacity of ~12 mmol g −1 under simulated flue gas conditions. The sorbent can be fully regenerated at low temperatures (below 100 °C) with relatively low energy consumption. The sorbent also exhibited good stability over repetitive adsorption–desorption cycling with regeneration in humid N 2 . Considering the versatility of the amine chemistry and the high amine content, as demonstrated in our model system, this method may provide new avenues for future development of CO 2 sorbents as well as other amine-functionalized systems, such as high-performance membranes, bioconjugates and basic catalysts. We note that the sorbent performance suffered, when a harsher regeneration protocol was used. The optimization of the amine molecular structure against oxidative degradation and the development of a more cost-effective, robust sorbent support should be targeted for further practical developments for this class of CO 2 sorbents. Synthesis of the sorbent Detailed synthesis for the sorbent is provided in Supplementary Methods . Briefly, the synthesis involves two major steps. First, a poly(2-methyl-2-oxazoline)/silica nanocomposite was synthesized via grafting-from cationic polymerization of oxazolines. 3-Iodopropyltrimethoxysilane functionalized silica support (0.8 g), 2-methyl-2-oxazoline, MeOX, (3.6 g) and benzonitrile (6 g) were mixed in a 50-ml rounded flask under dry N 2 and stirred at room temperature for 1 h. The mixture was then heated to 90 °C to initiate the cationic polymerization of MeOX. After polymerization at 90 °C for 120 h, the poly(MeOX)/silica nanocomposite was dispersed in water (30 g), filtered, washed with acetone and dried in a vacuum oven at 40 °C. In the second step, the dried nanocomposite (1.0 g) was hydrolysed in 50 ml of 5 M HCl aqueous solution at 90 °C for 24 h. The product was filtered, washed with acetone and redispersed in 50 ml of water. The pH of the dispersion was then adjusted to 10 using 1 M NaOH aqueous solution. The resulting PEI-tethered sorbent was filtered, washed subsequently with water and acetone and dried in a vacuum oven at 40 °C. Characterization TEM was conducted using a FEI TECNAI T12 Twin transmission electron microscope, operated at 120 kV. TEM specimens were prepared by placing a droplet of ethanol-diluted sample dispersion on a formvar-/carbon-coated microscope grid and dried in air. SEM was performed using a LEO 1550 FESEM operating between 0.5 and 3 kV. Elemental analysis of the sorbent samples was performed by Micro Analysis Inc. (Wilmington, DE). The dried samples were combusted in a pure oxygen environment. C, H and N analysis was based on the Pregl–Dumas method (CHN: ASTM D5291). XPS was performed on a SSX-100 spectrometer from Surface Science Instruments equipped with a monochromatic Al Kα X-ray source (hν=1,486.6 eV). Survey XPS spectra were acquired at 100 W with a pass energy of 150 eV over the range of 0–1,200 eV, with a resolution of 0.8 eV. The base pressure in the spectrometer was 3 × 10 −10 Torr during all measurements. All binding energies were referenced to the C 1s core level of C–C bonding at a binding energy of 285.0 eV. The high-resolution iodine spectrum was acquired with 11.75 eV pass energy, dwell time of 150 ms and averaged over 20 scans. FTIR spectrum of the sorbent was collected on a Bruker Optics Vertex80v vacuum FTIR spectrometer with 4 cm −1 resolution at room temperature. Solid-state cross-polarization magic-angle spinning 13 C NMR spectrum was obtained on a Bruker Avance 300 MHz spectrometer using the following parameters: 3,000 scans, a 90° pulse length of 5.2 μs and recycle times of 4 s. Inversely gated 13 C NMR of the cleaved polymer from the amine sorbent was recorded on a Bruker DRX-500 spectrometer at 50 °C (ref. 5 ). The sample was dissolved in D 2 O, and one drop of chromium acetylacetonate in deuterated dimethylsulfoxide was added. For each spectrum, 8,000 scans were collected with a relaxation time of 4 s. MALDI-TOF MS was performed on a Waters Micromass MALDI micro MX mass spectrometer equipped with a pulsed N 2 laser operating at 337 nm. 2,5-dihydroxybenzoic acid in CH 3 CN/H 2 O (v/v=50:50) was used as the matrix (25 mg ml −1 ). A water solution of the cleaved polymer (1 mg ml −1 ) was mixed with the matrix solution at a volumetric ratio of 1:1, of which 1 μl was spotted on the target plate. The MALDI-TOF MS spectra were recorded in linear, positive-ion mode and 50 spectra with each consisting of 10 laser shots were acquired for the sample. Nitrogen physisorption isotherms were measured at 77 K using a Micromeritics ASAP 2020 analyzer. The samples were degassed at 373 K under vacuum for 24 h. The specific surface areas of the samples were calculated by the BET method, using the adsorption data acquired at a relative pressure range of 0.05–0.25. The total pore volume was estimated from the amount of N 2 adsorbed at a relative pressure of 0.99. The pore size distributions of the samples were calculated from the analysis of the adsorption branch of the isotherm using the simplified Broekhoff-de Boer model. The heat changes during CO 2 adsorption and sorbent regeneration were estimated using a TA Q2000 DSC following the previously reported method [18] . The temperature and heat capacity measurements were calibrated using the melting point of indium and a sapphire crystal, respectively. In a typical measurement, about 6 mg of the sorbent was loaded in a Tzero aluminium pan and covered with a pan lid having a pinhole (~1 mm in diameter). The sample was heated to 100 °C and activated in humid N 2 (20 ml min −1 , relative humidity ~18% at 25 °C) for 30 min. The sample was then cooled down to 25 °C and equilibrated at that temperature for 10 more minutes. Subsequently, the gas was switched from N 2 to humid CO 2 (20 ml min −1 , relative humidity ~18% at 25 °C) and maintained at 25 °C for 60 min, after which the gas was switched back to humid N 2 and heated to 100 °C for sorbent regeneration. The apparent heat change caused by the gas switch was corrected using an empty Tzero aluminium pan with a pan lid. The reaction heat and the total energy penalty were calculated by integrating the heat flow during the adsorption and the desorption steps, respectively. CO 2 sorption measurements CO 2 adsorption studies were performed using a TA Instruments Q500 thermal gravimetric analyzer ( Supplementary Fig. 8 ). Humid 8% CO 2 (relative humidity ~18% at 25 °C) was used for the adsorption studies, and N 2 (relative humidity ~18% at 25 °C) was used as stripping gas for sorbent regeneration. In a typical adsorption process, about 5–10 mg of the sorbent was placed in a platinum sample pan. After being heated to 100 °C in humid N 2 (20 ml min −1 ) and held at that temperature for 30 min to remove the CO 2 adsorbed from the air, the sorbent was cooled down to 25 °C and equilibrated at that temperature for about 240 min. The gas was then switched to humid 8% CO 2 (20 ml min −1 ) at 25 °C for CO 2 adsorption. The capacity of the sorbent in mmol g −1 was calculated based on the weight gain of the sorbent during the adsorption step. After the adsorption step was completed, the gas was switched back to humid N 2 and the sorbent was regenerated at 100 °C. CO 2 adsorption in the packed bed was measured using the inline CO 2 analyzer system ( Supplementary Fig. 8 ). In a typical adsorption measurement, ~80 mg of the dried sorbent was dispersed on glass wool and packed in a quartz column (bed volume ~4 ml, internal diameter=0.7 cm and L=10 cm). N 2 and dilute CO 2 were humidified by passing the gases through a water bubbler at room temperature. The relative humidity of the gases was measured using a K-33 BLG relative humidity sensor (CO 2 Meter). Prior to CO 2 adsorption, the sorbent was activated at 100 °C for 1 h in humid N 2 (relative humidity ~18% at 25 °C) and then cooled down to room temperature. Subsequently, the inlet gas to the packed bed was switched to humid 8% CO 2 (relative humidity ~18% at 25 °C) with a flow rate of 45 ml min −1 . The CO 2 concentration of the effluent gas was monitored using a K-33 ICB CO 2 sensor (CO2Meter) with a sampling rate of ~2 s. Following adsorption for a certain time, the inlet gas to the packed bed was switched back to humid N 2 and the packed bed was heated to 100 °C for sorbent desorption. Following the same procedure, a blank control measurement was carried out using the bed packed only with glass wool to evaluate the dilution effect from gas changes. The CO 2 concentration profile after removal of the background was used for the sorbent capacity calculations. How to cite this article : Qi, G. et al . Sponges with covalently tethered amines for high-efficiency carbon capture. Nat. Commun. 5:5796 doi: 10.1038/ncomms6796 (2014).